Non-volatile electrically-driven repeatable magnetization reversal with no applied magnetic field Repeatable magnetization reversal under purely electrical control remains the outstanding goal in magnetoelectrics. Here we use magnetic force microscopy to study a commercially manufactured multilayer capacitor that displays strain-mediated coupling between magnetostrictive Ni electrodes and piezoelectric BaTiO 3 -based dielectric layers. In an electrode exposed by polishing approximately normal to the layers, we find a perpendicularly magnetized feature that exhibits non-volatile electrically driven repeatable magnetization reversal with no applied magnetic field. Using micromagnetic modelling, we interpret this nominally full magnetization reversal in terms of a dynamic precession that is triggered by strain from voltage-driven ferroelectric switching that is fast and reversible. The anisotropy field responsible for the perpendicular magnetization is reversed by the electrically driven magnetic switching, which is, therefore, repeatable. Our demonstration of non-volatile magnetic switching via volatile ferroelectric switching may inspire the design of fatigue-free devices for electric-write magnetic-read data storage. Magnetoelectric (ME) coupling [1] , [2] , [3] , [4] , [5] between ferroelectric and antiferromagnetic order has been demonstrated in multiferroic oxides, where a magnetic field can modify electrical polarization (TbMnO 3 , ref. 6 ; DyFeO 3 , ref. 7 ) or an electric field can modify antiferromagnetic order (BiFeO 3 ) [8] , [9] , [10] . There are few ferromagnetic piezoelectric materials [11] in which to attempt voltage-driven changes in magnetization, but the magnetization of thin ferromagnetic films may be electrically modified via strain from piezoelectric substrates (BaTiO 3 , refs 12 , 13 , 14 ; Pb(Mg 1/3 Nb 2/3 ) 0.72 Ti 0.28 O 3 , ref. 15 ; and Pb(Zr,Ti)O 3 , ref. 16 ); via exchange bias from ferroelectric-antiferromagnetic substrates either with (BiFeO 3 , ref. 17 ) or without (LuMnO 3 , ref. 18 ) possible strain assistance; via a gate that modifies semiconductor carrier concentration [19] ; or via the occupation of 3 d orbitals in ultra-thin Fe films [20] . Full reversals of global [12] , [18] , [19] , [21] and local [22] magnetization have been triggered via electrically controlled changes in carrier density [19] , orbital occupation [21] , strain [12] , [22] or exchange bias [18] . However, each magnetic reversal required an applied magnetic (driving) field to be set near the coercive field, such that the sign of this applied field had to be reversed for each magnetic reversal, cf. standard magnetic hysteresis loops. While we were completing this manuscript, anisotropic magnetoresistance data were presented [23] as evidence of electrically driven magnetic reversal in an island of Co 0.90 Fe 0.10 on BiFeO 3 , but this indirect measurement required an applied magnetic field whose possible unintended role in magnetization reversal cannot be ruled out, especially as the measurement field was similar to the coercive field. Therefore, magnetization reversal under purely electrical control with no applied magnetic field remains outstanding. This key goal in MEs is challenging because electric fields do not break time-reversal symmetry. Demonstrating electrical control of coercivity [19] , [24] , exchange bias [25] , [26] or magnetic anisotropy [20] , [27] is insufficient because, respectively, an electrically addressable coercivity is inextricably linked with an applied magnetic field; because exchange bias is an interfacial phenomenon that cannot readily drive magnetization reversal throughout a film of significant thickness; and because no new magnetic anisotropy axis can lie more than 90° from the anisotropy axis along which the local magnetization initially lies. It has been suggested that this latter challenge may be overcome by applying a suitable sequence of normal stresses near the pre-existing magnetic anisotropy axes of a small homogeneously magnetized Stoner-Wohlfarth particle [28] , [29] , but this has not been experimentally realised. In the opposite extreme of a highly inhomogeneous macroscopic ME system, we report the discovery of a feature with a nominally perpendicular magnetization that in zero applied magnetic field can be electrically reversed in a repeatable and non-volatile manner. This magnetic switching is experimentally indistinguishable from a full 180° magnetization reversal, but we suggest that the up and down magnetization states are slightly canted by a small in-plane magnetic field that is invariant and arises internally from the surrounding magnetic material. There is thus no violation of time-reversal symmetry. The large out-of-plane magnetization in the feature evidences a large out-of-plane uniaxial magnetic anisotropy that arises due to a large local in-plane stress. The reversal of this large out-of-plane magnetization, in the presence of the fixed in-plane field, is achieved by exploiting magnetization dynamics that are voltage- driven via a stress-induced reduction of the uniaxial out-of-plane anisotropy constant. The resulting changes in anisotropy field also depend on magnetization orientation, and, therefore, it is possible to achieve the key step of crossing the equatorial plane to reach a new equilibrium orientation below it. On subsequently removing the voltage, the out-of-plane anisotropy constant grows back to its original value, and, therefore, the magnetization is ultimately forced further below the equator until its out-of-plane component is eventually reversed with respect to its initial value. Characterization of multilayer capacitors We used poled multilayer capacitors (MLCs, Fig. 1a ) comprising polycrystalline magnetostrictive electrodes of Ni, and polycrystalline piezoelectric layers of doped BaTiO 3 (BTO). Similar MLCs show direct [30] and converse [31] strain-mediated ME coupling between these layers when measuring and applying voltages between the terminals, respectively. For energy-dispersive X-ray analysis (EDX) and magnetic force microscopy (MFM), MLCs were mechanically polished near the z direction to expose alternate Ni and BTO layers at the surface of an electrically inactive wedge ( Supplementary Fig. S1 ). MFM was performed near the thin end of this wedge (except in Supplementary Figs S2 and S3 ), with appropriate grounding to eliminate the possibility of spurious electrical contrast (Methods). EDX found no evidence of impurities in the Ni electrodes, except for an apparent contribution of 1.71 at.% Ti attributed to the juxtaposed BTO layers in which we found 3.21 at.% Zr. Scanning electron microscopy revealed that the Ni electrodes possess micron-scale structural features, which mimic the underlying grains of BTO ( Fig. 1b ), and are larger than the 20-40 nm Ni grains measured by X-ray diffraction. 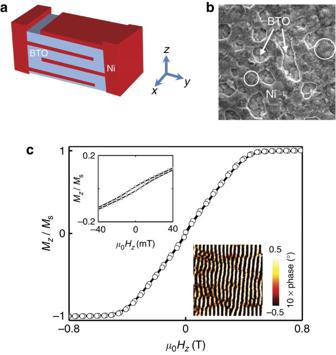Figure 1: MLC characterization. (a) MLC schematic, not to scale, showing 2 μm-thick Ni electrodes (red), and 6 μm-thick dielectric layers of doped BTO (blue). In reality, there are 200 Ni electrodes, and the assembly between MLC terminals is surrounded by doped BTO that lies below an outer polymer casing (not shown). MLCs were polished for scanning electron microscopy and MFM along the nominalzdirection. (b) Scanning electron microscopy image (30 μm × 30 μm) of polished MLC#1 after etching to expose sub-surface BTO. Circles indicate representative features in the Ni electrodes due to underlying BTO grains. For unpolished MLC#2 after poling, we show (c) hard-axis reduced magnetizationMz/Msas a function of applied fieldHz, at zero bias (○) and 200 V (solid line). Upper inset: detail of (c). Bottom inset: MFM image (30 μm × 30 μm) at magnetic remanence for the same MLC after polishing to reveal a near-surface electrode. Figure 1: MLC characterization. ( a ) MLC schematic, not to scale, showing 2 μm-thick Ni electrodes (red), and 6 μm-thick dielectric layers of doped BTO (blue). In reality, there are 200 Ni electrodes, and the assembly between MLC terminals is surrounded by doped BTO that lies below an outer polymer casing (not shown). MLCs were polished for scanning electron microscopy and MFM along the nominal z direction. ( b ) Scanning electron microscopy image (30 μm × 30 μm) of polished MLC#1 after etching to expose sub-surface BTO. Circles indicate representative features in the Ni electrodes due to underlying BTO grains. For unpolished MLC#2 after poling, we show ( c ) hard-axis reduced magnetization M z / M s as a function of applied field H z , at zero bias ( ○ ) and 200 V (solid line). Upper inset: detail of ( c ). Bottom inset: MFM image (30 μm × 30 μm) at magnetic remanence for the same MLC after polishing to reveal a near-surface electrode. Full size image The Ni electrodes in an unpolished MLC display shape anisotropy [31] with the hard-axis out-of-plane ( Fig. 1c ). The electrode saturation magnetization M s =290 kA m −1 is ~60% of the bulk value for Ni due to voids (nanocrystallinity forces only a 5% reduction [32] ). At remanence, a finite M z (upper inset, Fig. 1c ), and a regular pattern of weak stripe domains (bottom inset, Fig. 1c ), evidence a small perpendicular magnetic stress anisotropy ( Supplementary Note 1 ). An electric field that is large enough to produce strain-mediated changes of in-plane magnetization [31] had no discernible effect on out-of-plane magnetization M z ( Fig. 1c and Supplementary Fig. 3 ), but this does not preclude the local ME changes in M z that form the subject of this paper. Asymmetry due to tip-field reversal The Ni electrodes of polished MLCs contain a limited number of micron-scale magnetic features that we observed via a large MFM phase shift ( Fig. 2a ). Reversing the tip-field ( Fig. 2b ) reveals a pronounced asymmetry in the MFM signal ( Fig. 2c ) due to the influence of stray field from the magnetically hard tip on the softer feature magnetization. Quantitative analysis with MFM is challenging, but the peak-to-peak phase shift of ~4° ( Fig. 2c ) is so large that we are forced to conclude that the features comprise a single magnetic domain whose magnetization lies nominally out of the plane (under equivalent test conditions, our MFM test sample of metal-evaporated video tape from Digital Instruments shows a ~2° peak-to-peak phase shift due to stripe domains whose easy-axis magnetization lies 60° out of the plane [33] ). 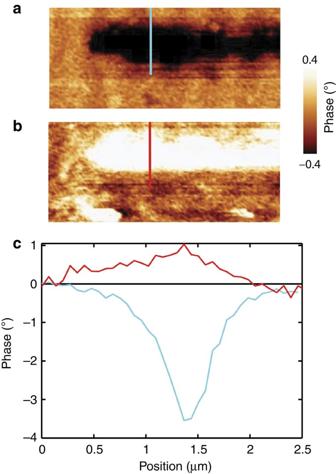Figure 2: MFM asymmetry due to tip-field reversal. MFM images (9 μm × 4 μm) for a region of nominally exposed Ni in MLC#3, (a) in zero electric field after having applied +200 V while at magnetic remanence, and (b) after subsequently reversing the tip-field. (c) Profiles along coloured lines in (a,b). This feature does not switch electrically. We were unable to perform equivalent tests on the switching feature ofFig. 3as the sample was destroyed by aggressive electrical testing.Supplementary Fig. S9shows atomic force microscopy images corresponding to (a,b). Figure 2: MFM asymmetry due to tip-field reversal. MFM images (9 μm × 4 μm) for a region of nominally exposed Ni in MLC#3, ( a ) in zero electric field after having applied +200 V while at magnetic remanence, and ( b ) after subsequently reversing the tip-field. ( c ) Profiles along coloured lines in ( a , b ). This feature does not switch electrically. We were unable to perform equivalent tests on the switching feature of Fig. 3 as the sample was destroyed by aggressive electrical testing. Supplementary Fig. S9 shows atomic force microscopy images corresponding to ( a , b ). Full size image ME features Applying and subsequently removing voltages to the terminals of polished MLCs created a limited number of additional magnetic features with out-of-plane magnetizations lying either parallel ( Supplementary Fig. S4 ) or antiparallel ( Supplementary Fig. S5 ) to the tip field. These applied voltages also resulted in various ME effects, which were volatile ( Supplementary Fig. S4 ), non-volatile ( Supplementary Fig. S2 ), repeatable ( Supplementary Fig. S6 ), and non-repeatable as seen at low ( Supplementary Fig. S7 ) and high ( Supplementary Fig. S8 ) magnification. The magnetic feature on which we focus here was remarkable because it underwent non-volatile electrically driven repeatable magnetic switching with no applied magnetic field ( Fig. 3a–d ). This switching is consistent with full (180°) magnetization reversal, as the large asymmetric MFM phase shifts ( Fig. 3e ) are similar to those seen on reversing the tip field when studying a single domain magnetized out-of-plane ( Fig. 2 ). However, we will model a more conservative scenario in which the up and down magnetization states are slightly canted by a fixed in-plane field from the surrounding and nominally invariant magnetic domains ( Fig. 3a–d ). 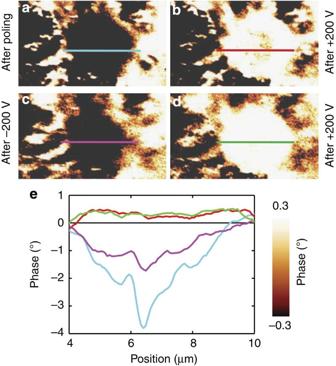Figure 3: Non-volatile electrically driven repeatable magnetization reversal with no applied magnetic field. Flattened MFM images (12 μm × 7 μm) for a region of nominally exposed Ni in MLC#4 at (a) magnetic remanence after poling, and subsequently in zero electric field after having applied (b) +200 V, (c) −200 V and (d) +200 V across MLC terminals. The reversals in the sign of the applied voltage are likely not significant as they do not alter the high-field strain31. (e) Profiles along coloured lines in (a–d). The corresponding atomic force microscopy images were unaffected by the electrical treatments (Supplementary Fig. S10). Figure 3: Non-volatile electrically driven repeatable magnetization reversal with no applied magnetic field. Flattened MFM images (12 μm × 7 μm) for a region of nominally exposed Ni in MLC#4 at ( a ) magnetic remanence after poling, and subsequently in zero electric field after having applied ( b ) +200 V, ( c ) −200 V and ( d ) +200 V across MLC terminals. The reversals in the sign of the applied voltage are likely not significant as they do not alter the high-field strain [31] . ( e ) Profiles along coloured lines in ( a – d ). The corresponding atomic force microscopy images were unaffected by the electrical treatments ( Supplementary Fig. S10 ). Full size image The nominally perpendicular magnetization and single-domain state of the feature ( Fig. 3 ) evidence a strong uniaxial z -axis anisotropy ( Supplementary Note 2 ), which arises due to isotropic in-plane stress σ >0 for Ni saturation magnetostriction <0. This local tensile stress in the feature arises following the release [34] of global in-plane compressive stress, that is, after applying and subsequently removing a voltage [31] . The magnetic discontinuity between the feature and the surrounding film may have a structural origin, as the lateral feature size is consistent with the topographical features seen after etching ( Fig. 1b ). Any such mechanical discontinuity would weaken interfacial exchange coupling, and we will assume that feature magnetization is only influenced by the surrounding film via a fixed in plane magnetic field, as discussed below. Electrically driven magnetization reversal in our single-domain Ni feature ( Fig. 3 ) is initiated when the voltage applied to the MLC terminals reduces K via a local reduction in σ that is large enough to exceed the global in-plane compressive stress observed in macroscopic measurements of strain [31] . This reduction in z -axis anisotropy could not modify the orientation of a purely z -axis magnetization, and we therefore assume slight canting due to a small invariant x -axis field H f from the surrounding magnetic domains in the same Ni layer. Therefore the feature magnetization M initially makes a small polar angle θ with respect to + z . When the voltage is applied, the stress-driven reduction in K reduces the magnitude of the z -axis anisotropy field H K , whose only component (2 K/μ 0 M s )cos θ depends on both K and θ . If the reduction in K were slow, then M would quasi-statically come to lie at the new equilibrium position above (rather than below) the equatorial x-y plane. However, if the reduction in K is sufficiently large and fast (see below), then it is possible for M to precess about H f + H K such that it settles at the new equilibrium position below the equatorial plane, with H K of reduced magnitude along − z . Following this key step of crossing the equatorial plane, the voltage may be removed at any time δ after reaching the new equilibrium. If the mechanical changes are reversible then K will return to its original value. Even if this increase in K is slow, M will rotate from the new equilibrium position below the equatorial plane until M z is reversed with respect to the starting configuration. The switched and unswitched states are energetically equivalent as H K is also switched. Therefore, the magnetic switching is repeatable. We will now present a quantitative model (Methods) for this Electrically driven coherent magnetic switching. The low-aspect-ratio feature ( Fig. 3 ) is treated as a sphere whose demagnetizing field does not influence magnetization direction (treating the feature as an ellipsoid would merely modify the values of K that we suggest below). We will investigate magnetic switching for two representative scenarios with μ 0 H f =100 mT ( Fig. 4a ) and μ 0 H f =10 mT ( Fig. 4b ), which are less than the μ 0 H f =200 mT of a spherical Lorentz cavity in Ni in order to account for the presence of both magnetic domains and voids around the feature. The initial and final anisotropy K hi must be large enough to produce a significant out-of-plane magnetization that is not reversed by the tip-field, and small enough to be significantly reduced by voltage-driven strain from the BTO lying immediately underneath the feature. We suggest that these criteria are simultaneously met for large changes in local strain that originate from 90° ferroelectric-domain switching, even if there is some degree of clamping. These changes in strain can be reversible [36] , [37] as required here, and domains can switch in as little as 1 ns (ref. 38 ) after exceeding the local switching field, regardless of the voltage sweep rate. We choose K hi =60 kJ m −3 to match the maximum possible change in anisotropy due to strain from BTO ( Supplementary Note 3 ) (2 K hi / μ 0 M s then corresponds to a flux density of 250 mT). 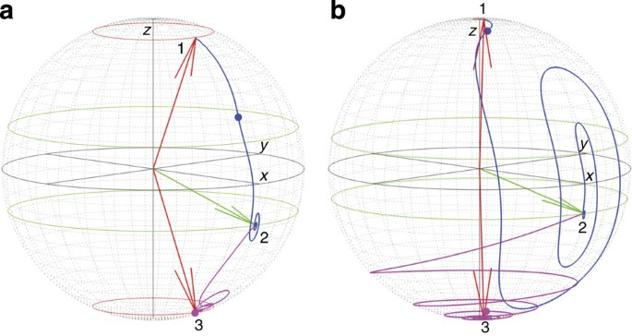Figure 4: Modelling of non-volatile Electrically driven repeatable magnetization reversal. The feature ofFig. 3is treated as a Ni macrospin whose magnetizationM(red arrow) makes angleθwith +z. It experiences both stress anisotropy field (0,0,(2K/μ0Ms)cosθ), and fixed magnetic field (Hf,0,0) from the surrounding magnetic domains. Assumingα=0.1 as measured for micron-sized Ni disks35, we investigate two representative scenarios with (a)μ0Hf=100 mT and (b)μ0Hf=10 mT. Voltage-driven stress reversibly reducesKover a ramp time of 1 ns fromKhi=60 kJ m−3to (a)Klo=25 kJ m−3and (b)Klo=2.45 kJ m−3. The two degenerate equilibrium-magnetization directions at zero (finite) voltage lie inx>0 at the intersections of thex-zplane and the red (green) circles, which are guides to the eye (the lower red circle in (b) is obscured).Minitially lies along (1) the zero-voltage equilibrium direction above thex-yplane. Our calculations show that it responds to the voltage-driven reduction ofKvia a trajectory (blue line, dot marks 1 ns ramp end) that takes it to (2) the finite-voltage equilibrium direction lying below thex-yplane after relaxation times of (a) 6.1 ns and (b) 40 ns. Subsequent removal of the voltage causesMto follow a trajectory (pink line, dot marks 1 ns ramp end) that takes it to (3) the zero-voltage equilibrium direction below thex-yplane, after a relaxation time that is 1.8 ns for both (a,b). The minimum total switching times (δ=0) obtained by adding the above relaxation times are (a) 7.9 ns and (b) 41.8 ns. A repeat of the temporary reduction inKwould recover initial magnetization direction (1). Video files corresponding to (a,b) appear as Supplementary Videos S1 and S2, respectively. Figure 4: Modelling of non-volatile Electrically driven repeatable magnetization reversal. The feature of Fig. 3 is treated as a Ni macrospin whose magnetization M (red arrow) makes angle θ with + z . It experiences both stress anisotropy field (0,0,(2 K / μ 0 M s )cos θ ), and fixed magnetic field ( H f ,0,0) from the surrounding magnetic domains. Assuming α =0.1 as measured for micron-sized Ni disks [35] , we investigate two representative scenarios with ( a ) μ 0 H f =100 mT and ( b ) μ 0 H f =10 mT. Voltage-driven stress reversibly reduces K over a ramp time of 1 ns from K hi =60 kJ m −3 to ( a ) K lo =25 kJ m −3 and ( b ) K lo =2.45 kJ m −3 . The two degenerate equilibrium-magnetization directions at zero (finite) voltage lie in x >0 at the intersections of the x-z plane and the red (green) circles, which are guides to the eye (the lower red circle in ( b ) is obscured). M initially lies along (1) the zero-voltage equilibrium direction above the x-y plane. Our calculations show that it responds to the voltage-driven reduction of K via a trajectory (blue line, dot marks 1 ns ramp end) that takes it to (2) the finite-voltage equilibrium direction lying below the x-y plane after relaxation times of ( a ) 6.1 ns and ( b ) 40 ns. Subsequent removal of the voltage causes M to follow a trajectory (pink line, dot marks 1 ns ramp end) that takes it to (3) the zero-voltage equilibrium direction below the x-y plane, after a relaxation time that is 1.8 ns for both ( a , b ). The minimum total switching times ( δ =0) obtained by adding the above relaxation times are ( a ) 7.9 ns and ( b ) 41.8 ns. A repeat of the temporary reduction in K would recover initial magnetization direction (1). Video files corresponding to ( a , b ) appear as Supplementary Videos S1 and S2, respectively. Full size image The initial orientation of M ((1) in Figs 4 and 5 ) is determined by the competition between H f along x , and H K along + z . When the voltage-driven stress reduces K from K hi to an appropriate value of K lo on a time scale of 1 ns, our calculations show that M undergoes damped precessional motion about H f + H K until it reaches the new equilibrium orientation below the x-y plane ((2) in Figs 4 and 5 ). On removing the voltage such that K grows back to K hi over 1 ns, M precesses once more until its z -axis component is reversed with respect to the starting configuration ((3) in Figs 4 and 5 ). Given that (2) in Figs 4 and 5 represents an equilibrium state, one may proceed to (3) after any delay δ , at the cost of time-wasting. For μ 0 H f =100 mT, one may switch | M z |~0.916 M s in 7.9 ns, using |Δ K |/ K hi ~60% consistent with some degree of local clamping ( Figs 4a and 5a ). For μ 0 H f =10 mT, one may switch a larger | M z |~0.999 M s in 41.8 ns, using |Δ K |/ K hi ~96% consistent with negligible local clamping ( Figs 4b and 5b ). Note that the 0.4 ns required for strain to propagate through a 2 μm Ni layer at the 5608, m s −1 speed of sound is negligible compared with the switching times reported here. 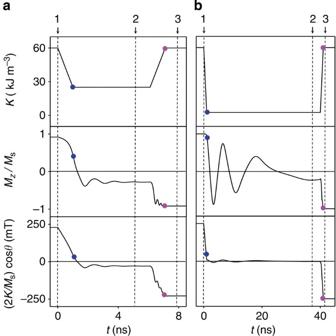Figure 5: Variations of anisotropy and out-of-plane magnetization during macrospin trajectories. For (a) and (b) inFig. 4, we plot the voltage-driven strain-mediated changes inK, and the resulting changes inMz/Ms, as functions of timet. We also plot the resulting and only component of the anisotropy field (2K/μ0Ms)cosθin terms of the corresponding flux density. Equilibrium positions 1, 2 and 3, and the blue and pink dots at ramp ends, correspond toFig. 4. Figure 5: Variations of anisotropy and out-of-plane magnetization during macrospin trajectories. For ( a ) and ( b ) in Fig. 4 , we plot the voltage-driven strain-mediated changes in K , and the resulting changes in M z / M s , as functions of time t . We also plot the resulting and only component of the anisotropy field (2 K / μ 0 M s )cos θ in terms of the corresponding flux density. Equilibrium positions 1, 2 and 3, and the blue and pink dots at ramp ends, correspond to Fig. 4 . Full size image For a range of values of damping-parameter α , we find that the critical step of switching from (1) to (2) in Figs 4 and 5 only occurs deterministically when the Electrically driven strain-mediated reduction in K forces the sign of M z ( t ) to undergo an odd number of changes before reaching equilibrium (pink regions in |Δ K | versus α phase diagrams, Fig. 6a ). By contrast, switching does not occur for an even number of such changes (blue regions, Fig. 6a ). Switching also fails to occur if M z ( t ) remains positive after ramping down K , that is, if |Δ K | is too small or if α is too large (black regions, Fig. 6a ). If |Δ K | is so high that H f ≥2 K lo / μ 0 M s , then the temporary reduction in K will drive the magnetization into the plane and parallel to H f , such that the return of K to K hi produces a final state whose out-of-plane magnetization is equally likely to be up or down (orange regions, Fig. 6a ). Supplementary Fig. S11 shows representative plots of M z ( t )/ M s for the pink, blue and black regions discussed above, with μ 0 H f =10 mT. It is attractive to use the smallest possible ramp times in order to increase the extent of switching regions in our phase diagrams ( Supplementary Fig. S12 ), but preliminary investigations show that any concomitant reduction in switching times is not necessarily significant. However, switching times may be reduced if the voltage is ramped down early to limit the time spent ringing near the intermediate magnetic configuration (that is, shortly before (2) in Figs 4a and 5a ). 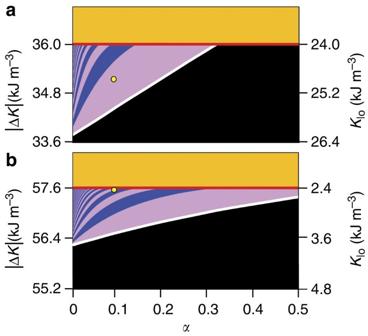Figure 6: Phase diagrams for non-volatile Electrically driven magnetization reversal. For (a)μ0Hf=100 mT and (b)μ0Hf=10 mT, a temporary reduction by |ΔK| fromKhi=60 kJ m−3toKloover a 1 ns ramp time, for a range of damping-parameter valuesα, yields switching (pink); no switching despite precession below thex-yplane (blue); precession above thex-yplane only and, therefore, no switching (black); and switching with 50% probability (orange). The yellow points in (a,b) correspond to (a,b) inFigs 4and5, respectively. Figure 6: Phase diagrams for non-volatile Electrically driven magnetization reversal. For ( a ) μ 0 H f =100 mT and ( b ) μ 0 H f =10 mT, a temporary reduction by |Δ K | from K hi =60 kJ m −3 to K lo over a 1 ns ramp time, for a range of damping-parameter values α , yields switching (pink); no switching despite precession below the x-y plane (blue); precession above the x-y plane only and, therefore, no switching (black); and switching with 50% probability (orange). The yellow points in ( a , b ) correspond to ( a , b ) in Figs 4 and 5 , respectively. Full size image In summary, we have experimentally demonstrated non-volatile Electrically driven repeatable magnetic switching that is consistent with full magnetization reversal ( Fig. 3 ). In contrast to previous reports, we require no externally applied magnetic field [12] , [18] , [19] , [21] , [22] , [23] . The resulting model permits nominally full reversal, and was inspired by recognizing that an Electrically driven strain-mediated fast and temporary reduction of uniaxial magnetic anisotropy can trigger precessional reversal of magnetization in the presence of a fixed transverse magnetic field. In both the experiment and the model, the sign of the magnetization can be repeatedly reversed from up to down, and down to up, using the same voltage-driven strain only, as the direction of the anisotropy field reverses when the sign of M z reverses. Overall, our work shows how to achieve magnetization reversal using voltage control of anisotropy. A magnetic field is also needed, but in contrast with previous schemes [12] , [18] , [19] , [21] , [22] , [23] , no changes in its direction or magnitude are required for repeatable switching. Our model based on a single macrospin may be exploited for high-density data storage with suitably designed nanomagnets, where the temporary reduction of anisotropy, and thus thermal stability, can be tolerated as the switching process is fast. The fixed magnetic field applied to many such nanomagnets could be provided by a single lithographically patterned element fabricated from a hard magnetic material. The anisotropy axis may be in the plane or out of the plane, for magnetic tunnel junctions or perpendicular magnetic recording media, respectively. The Electrically driven strain that controls the magnitude of the anisotropy may be either isotropic or uniaxial ( Supplementary Note 2 ). Alternatively, the anisotropy may be temporarily reduced using femtosecond laser pulses. Unlike competing mechanisms for fast magnetization reversal, we avoid the use of power-dissipating spin-torque currents, and changes in the control parameter need not be synchronised with precessional motion [39] as the intermediate state with the voltage on ((2) in Figs 4 and 5 ) is an equilibrium state. Samples We used KEMET 1210 MLCs poled in ~200 V. Polished MLCs could typically withstand repeated voltage cycles of amplitude 300 V, which corresponds to 500 kV cm −1 . Macroscopic measurements These were performed using a Philips diffractometer with CuK α radiation, and a Princeton Measurements Corporation vibrating sample magnetometer with electrical access to the sample [13] . Microscopic measurements of polished MLCs These were performed using a Philips XL30 SFEG for scanning electron microscopy, an Oxford Instruments spectrometer for EDX, and a Digital Instruments Dimension 3100 for atomic force microscopy and MFM. The MFM was performed at lift heights of 40–60 nm using low-moment ASYMFMLM Asylum Research tips of stiffness 2 N m −1 , coated with 15 nm of CoCr. The MFM tip-field was reversed by placing the tip and holder in μ 0 H =1 T along the tip axis. MFM tips were withdrawn ~1 mm before applying and then removing voltages for subsequent imaging at electrical remanence. The MFM tip and the electrode under study were grounded to minimize noise, and to avoid the possible influence of electric-field gradients in measurements away from electrical remanence ( Supplementary Fig. S4b only). MFM image analysis was performed using WSxM software [40] . Before MFM imaging, each polished and poled MLC was taken to magnetic remanence by applying and removing μ 0 H =1 T along the z -axis. The lateral extent of magnetic features could be estimated directly from MFM images because reversing tip magnetization ( Fig. 2 ) or feature magnetization ( Fig. 3 ) did not significantly modify apparent feature size. Magnetic changes that arise from Electrically driven strain at the lower interface of our 2 μm-thick Ni electrodes propagate to at least near the upper surface if detected by MFM, which probes to an estimated depth of 100-300 nm. Micromagnetic calculations A single Ni macrospin represented the uniform magnetization M of our switching feature ( Fig. 3 ), and we used in-house software with a 1 ps time step to execute a fourth-order Runge-Kutta integration of the Landau–Lifshitz–Gilbert (LLG) equation [41] : where γ is the gyromagnetic ratio for electrons; α is the effective damping parameter; and the feature is assumed to possess the bulk Ni saturation magnetization M s =480 kA m −1 . Effective field depends on the Gibbs free energy density G=− K cos 2 θ − μ 0 M·H f , which in turn depends on fixed magnetic field H f along hard-axis x , and uniaxial stress anisotropy field [42] H K along easy-axis z (uniaxial anisotropy constant K is under strain-mediated electrical control, , the magnitude and sign of H K is given by (2 K / μ 0 M s )cos θ , and μ 0 is the permeability of free space). The relaxation time for reaching equilibrium was estimated by determining the time t at which the maxima of the oscillating function |δ M z ( t )|/ M s fall below 10 −5 , where δ M z is the change per unit time step in the z -component of magnetization M z = M s cos θ . Our software permitted the anisotropy field to be modified during realistic 1–10 ns ramp times consistent with the speed of ferroelectric switching [38] . This is not possible using the commercially available LLG Micromagnetics Simulator, which we could, therefore, only use to confirm our results for an unrealistic 1 ps ramp time, which corresponds to the LLG time step ( Supplementary Fig. S13 ). How to cite this article: Ghidini, M. et al . Non-volatile Electrically driven repeatable magnetization reversal with no applied magnetic field. Nat. Commun. 4:1453 doi: 10.1038/ncomms2398 (2013).